Metabolic cross-feeding via intercellular nanotubes among bacteria Bacteria frequently exchange metabolites by diffusion through the extracellular environment, yet it remains generally unclear whether bacteria can also use cell–cell connections to directly exchange nutrients. Here we address this question by engineering cross-feeding interactions within and between Acinetobacter baylyi and Escherichia coli , in which two distant bacterial species reciprocally exchange essential amino acids. We establish that in a well-mixed environment E. coli , but likely not A. baylyi , can connect to other bacterial cells via membrane-derived nanotubes and use these to exchange cytoplasmic constituents. Intercellular connections are induced by auxotrophy-causing mutations and cease to establish when amino acids are externally supplied. Electron and fluorescence microscopy reveal a network of nanotubular structures that connects bacterial cells and enables an intercellular transfer of cytoplasmic materials. Together, our results demonstrate that bacteria can use nanotubes to exchange nutrients among connected cells and thus help to distribute metabolic functions within microbial communities. Microorganisms are ubiquitous on our planet and their metabolic activities significantly contribute to vital ecosystem processes [1] . In most cases, microbes exist in taxonomically diverse communities, whose structure is determined by a complex interplay between environmental factors and ecological interactions among its community members [2] , [3] . Strong selection pressures for limiting resources have resulted in the evolution of diverse strategies to survive and reproduce under these conditions and gave rise to the stunning richness of ecological interactions that can be observed within microbial communities [4] . Biotic interactions between two microorganisms can either positively or negatively affect the fitness of the interacting individuals. Negative fitness consequences can result from predation, parasitism or chemical warfare between microorganisms, while cooperative or mutualistic relationships can significantly benefit the strains involved [2] . Many of these interactions rely on either the active or passive release of chemical molecules into the environment [5] , [6] or, alternatively, a direct contact between bacterial cells [7] . In both cases, the spatial organization of a given microbial community dictates the outcome of these interactions [8] . For example, short distances between surface-attached cells facilitate the exchange of diffusible nutrients [9] and communication signals [10] . However, such a diffusion-based transfer of molecules between two cells bears a number of risks: unintended third parties may eavesdrop on the signal or consume the nutrient. Moreover, the exchanged molecule may degrade or be lost by a too fast diffusion [11] . To circumvent these problems, bacteria have evolved a multitude of different ways to directly deliver molecules to intended recipients. Such mechanisms include, for example, the production of outer membrane vesicles, as they are used by many bacterial species to deliver cargo to other cells [12] , [13] , [14] , [15] , [16] . Alternatively, bacterial cells may connect via channels [17] , nanotubes [18] , pili [19] or transiently fuse their outer membrane [20] to transfer cytoplasmic components or outer membrane materials. These direct cell–cell connections serve primarily three functions: first, genetic material such as plasmids is horizontally transferred between cells [12] , [21] , supplying the recipient with potentially beneficial genetic functions [22] , [23] . Second, chemical signals that help to coordinate social activities within microbial communities are trafficked between cells [16] . Third, proteins can be transferred between cells [18] , [20] , which are involved in social movement [14] or serve predatory bacteria as interspecific killing factors [15] . Another possibility, which remains virtually unexplored, is the utilization of intercellular connections to transfer nutrients between bacterial cells. While recent data suggest that significant proportions of the cytosol can be exchanged between connected cells [18] , clear experimental evidence for a possible nutritional function of the exchanged cytoplasmic constituents is lacking. Here we address this question by interrogating synthetically engineered cross-feeding interactions within and between the two bacterial species Acinetobacter baylyi and Escherichia coli . We establish that in a well-mixed environment E. coli , but likely not A. baylyi , can connect to other bacterial cells via membrane-derived, tubular structures (hereafter referred to as ‘nanotubes’) and use these to exchange cytoplasmic constituents. Furthermore, we show that cell attachment is demand-driven and contingent on the nutritional status of auxotrophic cells. Together, our results suggest that nanotubes can mediate the exchange of cytoplasmic nutrients among connected bacterial cells and thus help to distribute metabolic functions within microbial communities. Construction of synthetic cross-feeding interactions We engineered obligate cross-feeding interactions within and between A. baylyi and E. coli to achieve two main goals. First, genotypes should be unable to produce a certain amino acid and rely on an external supply of this metabolite for growth. Second, amino acid production levels should be sufficiently high to allow growth of a complementary cross-feeding genotype. To achieve this, two pairs of genes were deleted from the wild type (WT) background of both species: deleting the terminal genes of the histidine (His) and tryptophan (Trp) biosynthesis pathways hisD and trpB resulted in two ‘auxotrophs’ of both species unable to grow in the absence of an external supply of either His or Trp ( Supplementary Fig. 1 ). In addition, the regulatory regions of the His and Trp biosynthesis operons hisL (encodes the operon leader peptide) and trpR (encodes the tryptophan repressor protein) were deleted to eliminate negative transcriptional regulation of these two pathways, yielding two amino acid ‘overproducers’ (that is, genotypes impaired in the feedback control of amino acid production levels). Combining two deletion mutations (that is, ΔtrpB and ΔhisL ; ΔhisD and ΔtrpR ) in the same genetic background resulted in two ‘cross-feeders’ (that is, genotypes auxotrophic for one amino acid, which constitutively produce increased amounts of the other amino acid) with complementary metabolic requirements and amino acid production characteristics that allowed assembling four intra- and interspecific pairs of cross-feeders ( Fig. 1a ). Finally, each cross-feeding mutants was labelled with one of two plasmids that constitutively expressed either egfp or mCherry for subsequent differentiation. 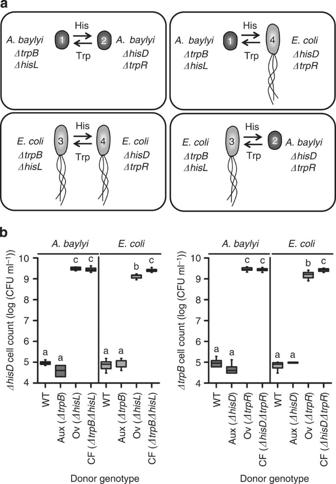Figure 1: Design of cross-feeding interactions and amino acid production levels of all genotypes. (a) Overview over all engineered cross-feeding interactions within and betweenAcinetobacter baylyiandEscherichia coli. Deletion ofhisDandtrpBrendered the resulting mutants auxotrophic for His and Trp, respectively, while deletion oftrpRandhisLincreased production levels of Trp and His, respectively. (b) Amino acid production of wild type (WT) and all generated mutant genotypes ofA. baylyi(dark-grey boxes) andE. coli(light-grey boxes) as determined by coculturing each donor genotype (xaxis) together with oneE. colibiosensor (initial ratio: 1:1) that was auxotrophic for either histidine (ΔhisD, left panel) or tryptophan (ΔtrpB, right panel). ‘Cell count’ refers to the number of biosensor cells that formed in coculture with a WT, auxotroph (Aux), amino acid overproducer (Ov) or cross-feeding genotype (CF) during 24 h. Values are colony-forming units (CFU) after 24 h minus the initial inoculum size. Different letters above boxes indicate significant differences between donor genotypes of both species (LSDpost hoctest:P<0.05,n=8). Figure 1: Design of cross-feeding interactions and amino acid production levels of all genotypes. ( a ) Overview over all engineered cross-feeding interactions within and between Acinetobacter baylyi and Escherichia coli . Deletion of hisD and trpB rendered the resulting mutants auxotrophic for His and Trp, respectively, while deletion of trpR and hisL increased production levels of Trp and His, respectively. ( b ) Amino acid production of wild type (WT) and all generated mutant genotypes of A. baylyi (dark-grey boxes) and E. coli (light-grey boxes) as determined by coculturing each donor genotype ( x axis) together with one E. coli biosensor (initial ratio: 1:1) that was auxotrophic for either histidine ( ΔhisD , left panel) or tryptophan ( ΔtrpB , right panel). ‘Cell count’ refers to the number of biosensor cells that formed in coculture with a WT, auxotroph (Aux), amino acid overproducer (Ov) or cross-feeding genotype (CF) during 24 h. Values are colony-forming units (CFU) after 24 h minus the initial inoculum size. Different letters above boxes indicate significant differences between donor genotypes of both species (LSD post hoc test: P <0.05, n =8). Full size image The His and Trp production levels of the enhanced green fluorescent protein (EGFP)-labelled variants of all newly constructed mutants and the WTs of both A. baylyi and E. coli were determined by coculturing each genotype together with one of two E. coli mutants auxotrophic for either His ( ΔhisD ) or Trp ( ΔtrpB ). Since the latter mutants require an external source of the focal amino acid to grow ( Supplementary Fig. 1 ), their growth in coculture is indicative of the amino acid production levels of the respective other strain [24] . Quantifying the amino acid production levels of all tested donors by determining the growth of cocultured auxotrophs (that is, number of colony-forming units (CFUs) formed during 24 h) revealed that overproducers and cross-feeders of both species produced His and Trp levels that significantly exceeded the production levels of both WTs and the corresponding other auxotrophs ( Fig. 1b ). Moreover, the corresponding overproducers and cross-feeders of both species supported the growth of cocultured auxotrophs to a similar extent ( Fig. 1b ), indicating that their amino acid production levels did not differ. Thus, the amino acid overproduction mutations (that is, ΔhisL , ΔtrpR ) significantly increased the His and Trp production levels of the corresponding mutants. Physical separation of strains prevents cross-feeding The newly designed cross-feeding genotypes were scrutinized for their ability to support the growth of a complementary partner of the same or the other species. Indeed, all cross-feeding mutants of E. coli grew in coculture with complementary E. coli cells, as well as cross-feeding A. baylyi genotypes ( Fig. 2a ). Surprisingly, the same cross-feeding mutants of A. baylyi that showed marked growth in coculture with E. coli exhibited virtually no growth when paired up with complementary genotypes of the same species ( Fig. 2a ). Next, we asked whether the transfer of amino acids between cross-feeders was based on the diffusion via the surrounding medium or whether a physical contact was required for cells to interact. To test this, the same coculture experiment was performed again, but this time bacterial populations were separated using a filter membrane ( Supplementary Fig. 2 ). For all combinations of cross-feeders tested, virtually no growth was detectable when the two bacterial populations were separated in this way ( Fig. 2a ). 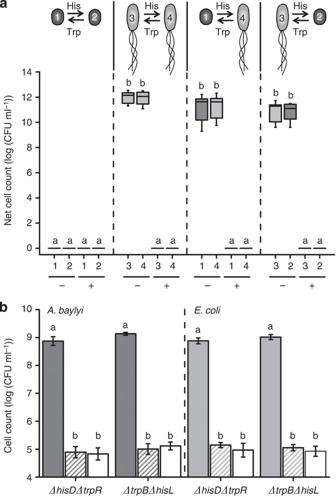Figure 2: Cross-feeding is contact-dependent. (a) Coculture experiments between all inter- and intraspecific cross-feeding interactions generated (genotype numbers and pictograms as inFig. 1a) in the absence (−) or presence (+) of a membrane filter that separated both populations to prevent a direct cell–cell contact (Supplementary Fig. 2), yet allowed passage of free amino acids (Supplementary Fig. 3). ‘Net cell count’ is the number of colony-forming units (CFU) a genotype reached in coculture during 24 h in minimal medium minus the CFU number reached in monoculture. Cytoplasmic markers (EGFP and mCherry) were swapped between cocultured genotypes. Each combination was replicated four times. (b) Growth of the cross-feeding genotypes at saturating concentrations of the required amino acid (that is, His or Trp, 100 μM, grey bars), a concentration of the required amino acid that significantly exceeded the amounts cross-feeding genotypes would have produced during 24 h of growth (that is, 0.5 μM, striped bars), or the absence of amino acids (white bars). ‘Cell count’ refers to the number of CFUs after 24 h minus the initial inoculum size. Mean values (±95% confidence interval) are shown. (a,b) Different letters indicate significant differences between groups (LSDpost hoctest:P<0.05,n=8). The two species are colour-coded asA. baylyi(dark grey) andE. coli(light grey). Figure 2: Cross-feeding is contact-dependent. ( a ) Coculture experiments between all inter- and intraspecific cross-feeding interactions generated (genotype numbers and pictograms as in Fig. 1a ) in the absence (−) or presence (+) of a membrane filter that separated both populations to prevent a direct cell–cell contact ( Supplementary Fig. 2 ), yet allowed passage of free amino acids ( Supplementary Fig. 3 ). ‘Net cell count’ is the number of colony-forming units (CFU) a genotype reached in coculture during 24 h in minimal medium minus the CFU number reached in monoculture. Cytoplasmic markers (EGFP and mCherry) were swapped between cocultured genotypes. Each combination was replicated four times. ( b ) Growth of the cross-feeding genotypes at saturating concentrations of the required amino acid (that is, His or Trp, 100 μM, grey bars), a concentration of the required amino acid that significantly exceeded the amounts cross-feeding genotypes would have produced during 24 h of growth (that is, 0.5 μM, striped bars), or the absence of amino acids (white bars). ‘Cell count’ refers to the number of CFUs after 24 h minus the initial inoculum size. Mean values (±95% confidence interval) are shown. ( a , b ) Different letters indicate significant differences between groups (LSD post hoc test: P <0.05, n =8). The two species are colour-coded as A. baylyi (dark grey) and E. coli (light grey). Full size image While significant growth occurred when the two cross-feeding mutants were exposed to saturating concentrations of His and Trp (that is, 100 μM), virtually no growth was detectable when cross-feeders were inoculated into unsupplemented minimal medium or minimal medium supplemented with 0.5 μM of either amino acid (that is, a concentration that exceeded the amount the corresponding intra- or interspecific counterparts would have released during 24 h, two- to fivefold, Supplementary Fig. 3 ) ( Fig. 2b ). This finding provided evidence that the amount of amino acids released by these mutants was not sufficient to explain the growth of cross-feeding genotypes in coculture ( Fig. 2a ). Moreover, an experiment to test whether His and Trp could freely pass through the filter membrane provided no evidence for the membrane acting as a diffusion barrier ( Supplementary Fig. 4 ). Together, these experiments established that cocultures of cross-feeding mutants among E. coli and between A. baylyi and E. coli showed a marked synergistic growth, which could not be explained by a release of His and Trp by cross-feeders into the extracellular environment, but instead required the physical presence of both partners in the same environment for cells to interact. Cross-feeding cells exchange cytoplasmic constituents An alternative to a diffusion-based transfer of amino acids through the external environment is direct cell–cell interactions that could enable the exchange of cytoplasmic amino acids among cells via, for example, nanotubes or pili. In such a case, other cytoplasmic constituents could be transferred to the respective other cross-feeding mutant along with the focal amino acids. To scrutinize this possibility, pairs of cross-feeding mutants within E. coli or between A. baylyi and E. coli were assembled and the cytoplasm of one partner (that is, the donor) was labelled with a plasmid that conferred resistance to the antibiotic ampicillin and constitutively expressed the fluorescent protein EFGP. In case of a cytoplasmic exchange among cells, both the plasmid and cytoplasmic protein might be transferred from the labelled donor to the previously unlabelled recipient cell. Transfer of plasmids was determined by plating dilutions of cocultures after 0 and 24 h on ampicillin-containing plates that were supplemented with either His or Trp to distinguish individual genotypes. Transfer of EGFP was assessed by quantifying the population-level proportion of cells that fluoresced in green colour at the onset of the experiment and after 24 h of coculture via flow cytometry. This experiment provided no support for a transfer of plasmids between cells under the given experimental conditions, since not a single colony formed on the corresponding antibiotic-containing plates. Although the proportion of plasmid-containing donor cells did not change significantly in any of the tested combinations during 24 h, a significant increase of EGFP-labelled cells during the same time implied that cytoplasmic protein was transferred from donor to recipient cells ( Fig. 3a ). Moreover, within the same combination of genotypes, EGFP was transferred from A. baylyi to E. coli and vice versa , thus indicating a bidirectional mode of transfer ( Fig. 3a ). 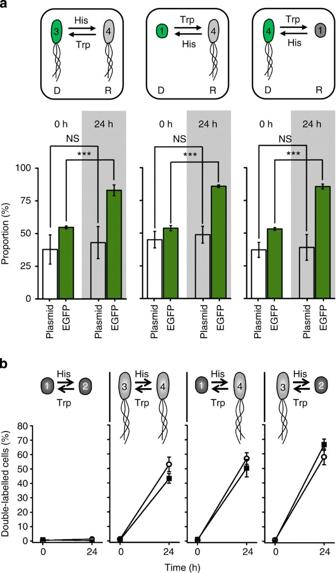Figure 3: Cross-feeding cells bidirectionally exchange cytoplasmic protein. (a) Two cross-feeding genotypes ofE. coliorA. baylyiandE. coliwere cocultured for 24 h. The donor (D) contained an EGFP-expressing plasmid that conferred resistance to the antibiotic ampicillin, while the recipient (R) was unlabelled. Shown is the mean proportion (±95% confidence interval) of all cells containing the labelling plasmid or the EGFP protein at the onset of the experiment (0 h) and after 24 h. Cell numbers were determined by plating on antibiotic-containing plates (plasmid presence) or flow cytometry (EGFP fluorescence emission). The proportion of plasmid-containing cells did not differ between time points (NS=not significant by a pairedt-test:P>0.05), while the proportion of EGFP-containing cells increased significantly during 24 h (pairedt-test: ***P<0.001). This experiment was replicated three times. (b) The cytoplasm of cross-feeding genotypes ofA. baylyiandE. coliwas labelled with plasmids expressing either EGFP or mCherry. The appearance of double-labelled cells (that is, containing both colours) in cocultures indicates a cytoplasmic exchange. Shown is the mean proportion (±95% confidence interval) of double-labelled cells after 0 and 24 h of growth in minimal medium, as determined by flow cytometry. This experiment was replicated eight times. Symbols represent the two possible arrangements of how markers were distributed among cross-feeders: mCherry/EGFP (circle) and EGFP/ mCherry (box). (a,b) Genotype pictograms like inFig. 1a. Figure 3: Cross-feeding cells bidirectionally exchange cytoplasmic protein. ( a ) Two cross-feeding genotypes of E. coli or A. baylyi and E. coli were cocultured for 24 h. The donor (D) contained an EGFP-expressing plasmid that conferred resistance to the antibiotic ampicillin, while the recipient (R) was unlabelled. Shown is the mean proportion (±95% confidence interval) of all cells containing the labelling plasmid or the EGFP protein at the onset of the experiment (0 h) and after 24 h. Cell numbers were determined by plating on antibiotic-containing plates (plasmid presence) or flow cytometry (EGFP fluorescence emission). The proportion of plasmid-containing cells did not differ between time points (NS=not significant by a paired t -test: P >0.05), while the proportion of EGFP-containing cells increased significantly during 24 h (paired t -test: *** P <0.001). This experiment was replicated three times. ( b ) The cytoplasm of cross-feeding genotypes of A. baylyi and E. coli was labelled with plasmids expressing either EGFP or mCherry. The appearance of double-labelled cells (that is, containing both colours) in cocultures indicates a cytoplasmic exchange. Shown is the mean proportion (±95% confidence interval) of double-labelled cells after 0 and 24 h of growth in minimal medium, as determined by flow cytometry. This experiment was replicated eight times. Symbols represent the two possible arrangements of how markers were distributed among cross-feeders: mCherry/EGFP (circle) and EGFP/ mCherry (box). ( a , b ) Genotype pictograms like in Fig. 1a . Full size image To determine whether all combinations of cross-feeding mutants exchange cytoplasmic protein in this way, all mutants of both species were labelled with plasmids constitutively expressing either EFGP or mCherry. The emergence of double-labelled cells during coculture—which would be indicative of a transfer of cytoplasm from one single-labelled cell to another one—was monitored by flow cytometry. This experiment demonstrated for all populations involving cross-feeding genotypes of E. coli that, already after 24 h of growth in shaken liquid culture, more than 50% of all cells within these populations were simultaneously labelled with both EGFP and mCherry ( Fig. 3b ; Supplementary Fig. 5a–h ). Extending the time of coculture until 48 h even resulted in more than 60% of all cells being simultaneously labelled with both fluorescent proteins ( Supplementary Fig. 5a–h ). In contrast, virtually no double-labelled cells (that is, <2%) could be detected in cross-feeding consortia consisting exclusively of A. baylyi ( Fig. 3b ; Supplementary Fig. 5a,b ). Repeating the same experiment with a more fine-grained temporal resolution provided evidence for double-labelled cells already 12 and 15 h after the onset of the experiment ( Supplementary Fig. 5i–k ). A striking link between the increase in productivity of cross-feeding consortia and the formation of double-labelled cells over time bolstered the interpretation that growth of these cultures was indeed contingent on direct cell–cell interactions ( Supplementary Fig. 5i–k ). The observation that populations of mCherry-labelled cells consistently declined much faster than cocultured EGFP-labelled cells ( Supplementary Fig. 5 ) could be explained with significantly increased fitness costs incurred by the mCherry -containing plasmid relative to its EGFP-expressing counterpart ( Supplementary Fig. 6 ). Cultivating monocultures of A. baylyi and E. coli cross-feeders that contained either the mCherry- or the EGFP-expressing plasmid for 48 h and determining emission levels of both red and green fluorescence after 0, 24 and 48 h by flow cytometry corroborated that all cultures analysed emitted light exclusively at the expected wavelength over the entire experimental period ( Supplementary Fig. 7 ). Thus, this experiment ruled out that the previously observed emergence of double-labelled cells was due to the emission of both colours from single-labelled cells. However, a cell that is scored as emitting both green and red fluorescence in the flow cytometer may also result from the physical attachment of two differentially labelled cells, rather than an exchange of cytoplasmic protein. However, three lines of evidence support the interpretation that indeed single cells contained both fluorescent proteins: first, dissociating possible cell clumps by vortexing did not significantly reduce the number of double-labelled cells ( Supplementary Fig. 8a ). Even treatment with a commercially available cell dissociation solution reduced the number of double-labelled cells by 19 and 11% only in the within- E. coli cocultures, while it did not affect the number of double-labelled cells in any of the interspecific cocultures ( Supplementary Fig. 8a ). Second, the size distribution of double-labelled cells determined as the forward scatter (FSC) in the flow cytometer [25] was congruent with the size distribution of EGFP-labelled WT cells of E. coli . Third, analysing cocultures of pairwise cross-feeding consortia within E. coli or between A. baylyi and E. coli under the fluorescence microscope revealed individual cells that fluoresced in both red and green colour ( Fig. 4c ). 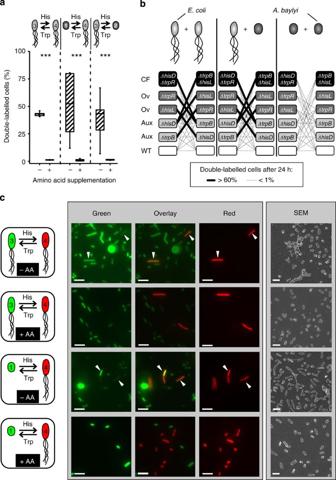Figure 4: Transfer of cytoplasmic markers depends on amino acid availability. (a) Proportion of double-labelled cells as determined by flow cytometry in cocultures of cross-feeding genotypes after 24 h of growth in the absence (−) or presence (+) of the required amino acids His and Trp (100 μM each). Pairedt-test: ***P<0.001. This experiment was replicated eight times. (b) Proportion of double-labelled cells formed in pairwise coculture experiments of differentially labelled wild type (WT), auxotrophs (Aux), amino acid overproducers (Ov), or cross-feeding genotypes (CF). Number of double-labelled cells after 24 h was determined by flow cytometry. This experiment was replicated four times. (c) Four representative pairs of cross-feeding interactions withinE. coli(rows 1 and 2) or betweenA. baylyiandE. coli(rows 3 and 4) were cocultured in the absence (rows 1 and 3) or presence (rows 2 and 4) of the two required amino acids (AAs) His and Trp (100 μM each). Fluorescence pictures show cells labelled with EGFP (green), mCherry (red) or both markers simultaneously (overlay). Scale bars, 5 μm. White triangles highlight cells where transfer occurred. The last column shows scanning electron micrographic (SEM) images of the corresponding cocultures. Scale bars, 2 μm. Figure 4: Transfer of cytoplasmic markers depends on amino acid availability. ( a ) Proportion of double-labelled cells as determined by flow cytometry in cocultures of cross-feeding genotypes after 24 h of growth in the absence (−) or presence (+) of the required amino acids His and Trp (100 μM each). Paired t -test: *** P <0.001. This experiment was replicated eight times. ( b ) Proportion of double-labelled cells formed in pairwise coculture experiments of differentially labelled wild type (WT), auxotrophs (Aux), amino acid overproducers (Ov), or cross-feeding genotypes (CF). Number of double-labelled cells after 24 h was determined by flow cytometry. This experiment was replicated four times. ( c ) Four representative pairs of cross-feeding interactions within E. coli (rows 1 and 2) or between A. baylyi and E. coli (rows 3 and 4) were cocultured in the absence (rows 1 and 3) or presence (rows 2 and 4) of the two required amino acids (AAs) His and Trp (100 μM each). Fluorescence pictures show cells labelled with EGFP (green), mCherry (red) or both markers simultaneously (overlay). Scale bars, 5 μm. White triangles highlight cells where transfer occurred. The last column shows scanning electron micrographic (SEM) images of the corresponding cocultures. Scale bars, 2 μm. Full size image Taken together, these results show that cross-feeding cells can bidirectionally exchange cytoplasmic constituents such as protein, yet they provided no evidence for a transfer of plasmid DNA (that is, pJBA24) between cells. Cytoplasmic exchange depends on nutritional status of cells Since both cross-feeding genotypes vitally required one amino acid to grow, we hypothesized that externally adding the focal amino acid to the growth environment should abolish the experimentally imposed obligate requirement for cross-feeding. As a consequence, these conditions should also eliminate the exchange of cytoplasmic markers such as EGFP and mCherry among cross-feeders. An experiment to test this hypothesis clearly validated that the transfer of cytoplasmic constituents was governed by the physiological demand for amino acid cross-feeding: after 24 h, cocultures of cross-feeding consortia that consisted of either two E. coli mutants or A. baylyi and E. coli exhibited a population-level ratio of double-labelled cells of around 40% when grown in unsupplemented minimal medium. In contrast, when the growth medium was supplemented with His and Trp, the proportion of double-labelled cells reached less than 1.4% of the total population ( Fig. 4a ), thus indicating that the exchange of cytoplasmic constituents was driven by the nutritional status of an E. coli cell. Similarly, no double-labelled cells could be detected by fluorescence microscopy when cocultures of cross-feeding genotypes were supplemented with His and Trp ( Fig. 4c ). Finally, coculture experiments between all possible combinations of differentially labelled WTs, auxotrophs, overproducers, and cross-feeders of both species revealed two conditions for a cytoplasmic exchange to be detectable by flow cytometry ( Fig. 4b ). First, one of the two partners needed to carry a mutation causing amino acid overproduction. Second, the respective other cells needed to be an E. coli cell auxotrophic for the corresponding amino acid. Altogether, this set of experiments revealed that the species-specific exchange of cytoplasmic constituents between two bacterial cells was driven by the physiological demand for a given amino acid, as well as the presence of other cells satisfying this need. Cytoplasmic exchange requires the mixing of cocultures All experiments so far have been conducted under shaken environmental conditions. A static incubation of cocultures, however, could enhance the exchange of cytoplasmic constituents due to facilitated cell–cell interactions under non-disturbed conditions. This hypothesis was tested by incubating cross-feeding consortia consisting of one (that is, E. coli ) or both species under static or continuously shaken environmental conditions, and quantifying the proportion of double-labelled cells after 0 and 24 h by flow cytometry. In contrast to expectations, this experiment clarified that the shaking of cultures was essential for a cytoplasmic exchange to take place ( Supplementary Fig. 9 ). Under shaking conditions, around 50% of cells were double-labelled after 24 h of growth, while almost no double-labelled cells emerged when cocultures were incubated under static conditions ( Supplementary Fig. 9a,c,e ). The lacking cytoplasmic exchange under static incubation conditions strikingly coincided with a severely reduced growth of these cultures ( Supplementary Fig. 9b,d,f ) relative to cocultures that were incubated under shaken conditions, thus corroborating that an exchange of cytoplasmic material was essential for growth of these obligate cross-feeders. In contrast to our expectations, this experiment indicated that the shaking of cultures promoted the exchange of cytoplasmic constituents. Cells connect via membrane-derived nanotubes What is the structural basis for the observed transfer of cytoplasmic elements among cross-feeding cells? To answer this question, scanning electron micrographs of cross-feeding consortia consisting of either E. coli or A. baylyi and E. coli were recorded. In the presence of amino acids (that is, His and Trp, 100 μM each), cocultures of cross-feeding genotypes grew as individual cells with no discernible sign of a physical attachment of two or more cells ( Fig. 4c ). However, without an external supply of His and Trp, cells of both types of cocultures consistently formed tubular structures that connected cells ( Figs 4c and 5 ). The average diameter of these nanotubes was 80±10 nm, and the distance covered between two cells ranged between 0.05 and 14 μm. 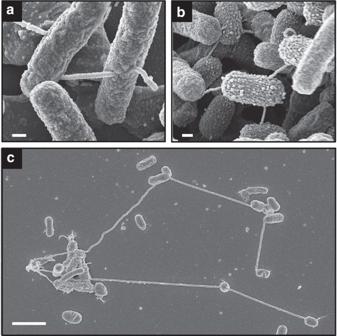Figure 5: Nanotubular structures connect cross-feeding cells. Intercellular connections form between two cross-feeding genotypes ofE. coli, as well as betweenA. baylyi and E. coli.Shown are scanning electron micrographic images of (a) anE. coli ΔtrpBΔhisLandE. coli ΔhisDΔtrpRcoculture after 24 h, as well as (b,c) anA. baylyi ΔhisDΔtrpRandE. coli ΔtrpBΔhisLcoculture after (b) 48 h and (c) 24 h of growth in unsupplemented minimal medium. Scale bars, 0.2 μm (a,b), 2 μm (c). Figure 5: Nanotubular structures connect cross-feeding cells. Intercellular connections form between two cross-feeding genotypes of E. coli , as well as between A. baylyi and E. coli. Shown are scanning electron micrographic images of ( a ) an E. coli ΔtrpBΔhisL and E. coli ΔhisDΔtrpR coculture after 24 h, as well as ( b , c ) an A. baylyi ΔhisDΔtrpR and E. coli ΔtrpBΔhisL coculture after ( b ) 48 h and ( c ) 24 h of growth in unsupplemented minimal medium. Scale bars, 0.2 μm ( a , b ), 2 μm ( c ). Full size image To identify whether these intercellular connections consist of membrane-derived lipids, 9-h-old interspecific cocultures of the cross-feeding mutants A. baylyi ΔhisDΔtrpR and E. coli ΔtrpBΔhisL were labelled with the lipophilic dye DiO that intercalates in lipid membranes [20] . Subsequent in vivo fluorescent imaging of the otherwise mCherry-labelled cells should pinpoint the potential lipid-based nature of extracellular appendages by their green fluorescence. In line with these expectations, the lipophilic dye stained threads that connected multiple cells, indicating they consist of membrane-derived lipids ( Fig. 6 ). 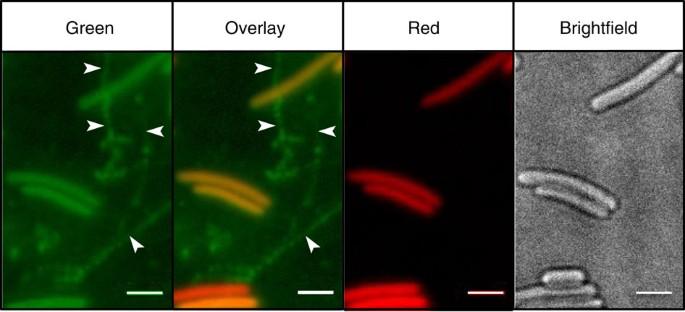Figure 6: Nanotubes consist of membrane-derived lipids. Cocultures of cross-feeding genotypes ofA. baylyi ΔhisDΔtrpRandE. coli ΔtrpBΔhisL(both mCherry labelled) after 9 h of growth were stained with a lipophilic dye (DiO) that intercalates in membranes. Lipid membranes fluoresce in green colour. Pointers indicate nanotubes that connect cells. Scale bars, 2 μm. Figure 6: Nanotubes consist of membrane-derived lipids. Cocultures of cross-feeding genotypes of A. baylyi ΔhisDΔtrpR and E. coli ΔtrpBΔhisL (both mCherry labelled) after 9 h of growth were stained with a lipophilic dye (DiO) that intercalates in membranes. Lipid membranes fluoresce in green colour. Pointers indicate nanotubes that connect cells. Scale bars, 2 μm. Full size image Finally, imaging consortia of cross-feeding mutants of A. baylyi ( ΔhisDΔtrpR containing pJBA24- mCherry ) and E. coli ( ΔtrpBΔhisL labelled with pJBA24- egfp ) by fluorescence microscopy clearly showed that nanotubes fluoresced in green colour ( Fig. 7a,b ), implying they are hollow and contained EGFP. Next, time-lapse fluorescence microscopy experiments were set up to visualize transfer of cytoplasmic material using the same interspecific pair of cross-feeding mutants. However, nanotubes did not establish when cross-feeding genotypes were cocultured on agarose pads. Instead, when cells were allowed to form nanotubes in a shaken, liquid culture and subsequently transferred to agarose pads, we observed a striking example for a cytoplasmic transfer via nanotubes: a dividing mCherry-labelled cell (most likely A. baylyi) that was connected to several EGFP-labelled cells (most likely E. coli ) via green-fluorescing nanotubes displayed a continuous, yet moderate increase in its green fluorescence levels over 32 min ( Fig. 7b,c ; Supplementary Movie 1 ). Then, within 2 min, the intensity of green fluorescence jumped from 113±11 to 455±34 arbitrary fluorescence units ( Fig. 7c ). This stark increase in green fluorescence during such a short time is unlikely to be caused by an increased EGFP expression level, thus further supporting that protein but not plasmids are transferred between cells. Control measurements from the same images of five randomly chosen mCherry- and EGFP-labelled cells that only showed fluorescence in their respective channel and which were not visibly connected to any other cell ( Fig. 7d,e ) ruled out that the previously observed increase in green fluorescence was due to stochastic fluctuations. These findings strongly suggest the involvement of nanotubes in mediating the observed intercellular transfer of cytoplasmic constituents. 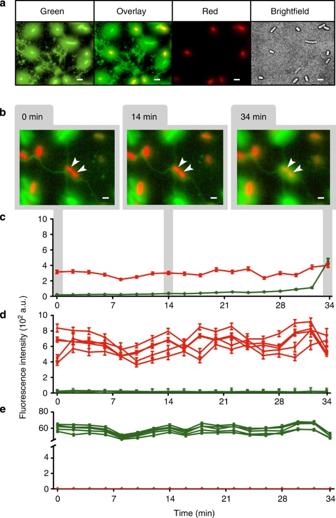Figure 7: Nanotubes transport cytoplasmic constituents. Cocultures of cross-feeding genotypes ofA. baylyi ΔhisDΔtrpR(mCherry labelled) andE. coli ΔtrpBΔhisL(EGFP labelled) after 9 h of growth. (a) Fluorescence and brightfield microscopic images show a network of nanotubes and vesicles that contain EGFP. Scale bars, 4 μm. (b) Fluorescence time-lapse microscopy reveals an increase in green fluorescence in a dividing mCherry-labelled cell (pointers) over time. The focal cells are attached to an EGFP-containing nanotube that projects to several EGFP-containing cells. Scale bars, 2 μm. (c–e) Change in red (red lines) and green (green lines) fluorescence intensity (102arbitrary units (a.u.)) over time. Values for each time point were derived by analysing cells on the same microscopic field. Points are means (±95% confidence interval) of 30 longitudinal measurements per cell with background fluorescence levels subtracted. Background fluorescence varied marginally over time (95% confidence intervals of green fluorescence: ±2.9 a.u., red fluorescence: ±1.8 a.u.). Shown is the change in fluorescence levels of (c) the focal cells highlighted inb, (d) five randomly chosen mCherry-containing cells, and (e) five randomly chosen EGFP-containing cells. The transfer event shown inbandcis the same as that depicted inSupplementary Movie 1(unprocessed images are available at the Dryad Digital Repository,http://doi.org/10.5061/dryad.ds68k). Figure 7: Nanotubes transport cytoplasmic constituents. Cocultures of cross-feeding genotypes of A. baylyi ΔhisDΔtrpR (mCherry labelled) and E. coli ΔtrpBΔhisL (EGFP labelled) after 9 h of growth. ( a ) Fluorescence and brightfield microscopic images show a network of nanotubes and vesicles that contain EGFP. Scale bars, 4 μm. ( b ) Fluorescence time-lapse microscopy reveals an increase in green fluorescence in a dividing mCherry-labelled cell (pointers) over time. The focal cells are attached to an EGFP-containing nanotube that projects to several EGFP-containing cells. Scale bars, 2 μm. ( c – e ) Change in red (red lines) and green (green lines) fluorescence intensity (10 2 arbitrary units (a.u.)) over time. Values for each time point were derived by analysing cells on the same microscopic field. Points are means (±95% confidence interval) of 30 longitudinal measurements per cell with background fluorescence levels subtracted. Background fluorescence varied marginally over time (95% confidence intervals of green fluorescence: ±2.9 a.u., red fluorescence: ±1.8 a.u.). Shown is the change in fluorescence levels of ( c ) the focal cells highlighted in b , ( d ) five randomly chosen mCherry-containing cells, and ( e ) five randomly chosen EGFP-containing cells. The transfer event shown in b and c is the same as that depicted in Supplementary Movie 1 (unprocessed images are available at the Dryad Digital Repository, http://doi.org/10.5061/dryad.ds68k ). Full size image Altogether, these analyses established that cross-feeding cells exchanged cytoplasmic constituents via an intercellular network of nanotubular structures that consisted of membrane-derived lipids. Cooperative metabolic interactions are very common among both Archaea and Bacteria [6] , [26] and these ‘syntrophic’ interactions are in many cases vitally important for the fitness of the microbes involved. However, since the exchanged commodities are often costly to produce, a diffusion-based transfer between cells via the extracellular environment entails risks: the metabolite may be lost or be consumed by an unintended third party. This problem even aggravates in agitated, aqueous ecosystems, where released compounds diffuse at high rates, thus hampering the build-up of sufficiently high local concentrations. Our results demonstrate that E. coli can solve this problem by employing cell–cell connections for a targeted transfer of cytoplasmic constituents. Utilizing engineered obligate cross-feeding interactions, we show that (i) E. coli , but likely not A. baylyi , can exchange nutrients and proteins in a contact-dependent manner with cells of the same or a different species ( A. baylyi ), (ii) the observed exchange was bidirectional and required a mixing of cocultures, (iii) lipid-based nanotubes were the structural basis for the observed cytoplasmic exchange, and (iv) the establishment of intercellular bridges and the exchange of cytoplasmic materials was strongly dependent on the nutritional status of a given cell. As such, our study provides first experimental evidence for an intercellular transfer of nutrients via nanotubes. The observation that E. coli established tubular connections with other bacterial cells is strikingly reminiscent of Myxococcus xanthus [15] , [27] cells, which have been shown to form a discrete, three-dimensional network of membrane tubes that interconnects cells. Cells of this social bacterium use membrane extensions to mediate the intercellular transfer of outer membrane proteins and lipids [14] , yet not cytoplasmic contents [27] . Given the recent evidence that Bacillus subtilis cells can exchange cytoplasmic elements such as protein and plasmid DNA via tubular connections [18] , it is tempting to speculate that this type of contact-dependent metabolite exchange may be more common in bacteria than previously thought. Many bacteria [28] , [29] , including E. coli [12] , are known to produce membrane vesicles that are involved in an intercellular transport of chemical signals [16] , lipids [30] , protein [31] , and DNA [12] , as well as in promoting adherence to other bacterial or eukaryotic host cells [32] , [33] . In most of these cases, membrane vesicles are believed to pinch off the producing cell and traverse the external environment as cell-independent units that eventually fuse with potential recipients [16] . Also in our experiments we observed vesicular structures that appeared attached to bacterial cells or seemingly free-floating in the cell external environment ( Fig. 7a,b ). While the results of the population separation experiment ( Fig. 2a ) and the fluorescence microscopic analyses are inconsistent with the idea that cytoplasmic elements were trafficked with free membrane vesicles, their functional role in our experiments remains elusive. Currently, we are working on identifying the structural basis of nanotube formation and elucidating the potential involvement of membrane vesicles in this process. The results of this analysis will be reported elsewhere. What triggered the formation of nanotubes in our experiments? Deleting key steps of amino acid biosynthetic pathways likely rendered the resulting E. coli mutants starving for His and Trp [34] . This experimentally induced nutrient limitation represents a strong stimulus [35] that could have triggered the observed response. Accordingly, both the transfer of cytoplasmic markers between cells ( Fig. 4a ) and the formation of nanotubes ( Fig. 4c ) could be effectively prevented by supplementing the growth medium with the two focal amino acids. These findings imply the existence of a regulatory mechanism, which, depending on the degree of nutrient starvation, activates the nanotube-mediated cell attachment in E. coli to remedy shortcomings for the required metabolites. In our study, cross-feeding E. coli cells could both serve as donor and recipient of amino acids ( Fig. 2a ) and protein ( Figs 3 and 4 ), suggesting the exchange of cytoplasmic constituents was bidirectional on a population level. A bidirectional exchange of cytoplasmic elements has been previously documented in B. subtilis cells that exchanged plasmids and cytoplasmic protein via nanotubes [18] , as well as in archaea [36] , [37] that use cytoplasmic bridges to reciprocally exchange non-conjugative plasmids between cells. Strikingly, the labelling plasmid used in this study (pJBA24) was not transferred between cells, which could imply the plasmid was bound to the host’s chromosome and/or its inner membrane [38] . Future work should investigate whether other plasmids that differ in, for example, their copy number or mode of replication/segregation can be exchanged in this way. Finally, the degree of specificity with which cytoplasmic elements can be exchanged between cells remains unknown. In particular, an uncontrolled passage of regulatory or catalytic elements through nanotubes may jeopardize homeostasis and development of connected cells. Thus, it will be interesting to explore whether nanotube-forming bacteria utilize diffusion barriers [39] or specialized secretion systems [40] to selectively control nanotube traffic. In this study, a passive movement was required for cell–cell connections to successfully establish ( Supplementary Fig. 9 ). A possibility to account for this observation is that outgrowing nanotubes might have impaired the active swimming motility of cells. Given the length nanotubular structures can reach (that is, up to 14 μm, Figs 5c and 7b ), it seems likely that these appendages impede swimming. As a consequence, physical mixing of cells was required to increase the chance of a given recipient to encounter and attach to suitable donor cells. This is in contrast to previous reports on B. subtilis [18] or M. xanthus [27] , [41] in which cell–cell interactions required a solid surface. In our experiments, nanotubes did not establish on (agarose) surfaces. Even when cells were allowed to pre-form nanotubes in liquid cultures and then were transferred to an agarose pad, nanotubes were only transiently visible and then appeared to destabilize over time. To successfully attach to other bacterial cells in an agitated, liquid environment, E. coli needed not only to be able to recognize suitable cells, but also required an efficient mechanism to capture detected cells. In our experiments, amino acids released from cross-feeding genotypes could have served as a chemical cue to recognize suitable host cells [42] , [43] , [44] . However, it remains unclear whether E. coli utilizes chemosensory mechanisms to specifically identify target cells or whether the binding of nanotubes is rather promiscuous. Our finding that E. coli readily accepted A. baylyi as a suitable host suggests metabolic suitability rather than kin discrimination mechanisms [45] governed the choice of E. coli . Identifying the molecular mechanisms that regulate the attachment of two bacterial cells as well as degree of specificity that underlies this process are exciting areas of research that should be addressed in the future. Starving cells that were part of the intercellular network ‘imported’ certain metabolites, while other cells functioned as a source for the required compounds. Depending on the net benefit incurred to the cells involved, the spectrum of possible ecological interactions that could result from this attachment process ranges from truly parasitic, where mainly the receiver benefits, to mutualistic interactions, in which both parties benefit [46] . Although in this study the ecological interactions were synthetically contrived, the observation that E. coli but not A. baylyi was capable of satisfying its metabolic requirements by connecting itself to other bacterial cells was not experimentally arranged. The discovery that the loss of conditionally essential biosynthetic genes induced the formation of nanotubes ( Fig. 4 ) represents a previously unknown strategy of E. coli that may help starving cells to survive in their natural environment. Given the widespread occurrence of pili, nanotubes, or other mechanisms bacteria utilize to exchange molecules, the intentional or enforced establishment of intercellular connections to engage in cooperative and parasitic nutritional interactions may represent a common ecological strategy pursued by bacteria. One of the best-studied examples of a metabolic parasitism involves two species of archaea: Nanoarchaeum equitans grow attached to the surface of Ignicococcus hospitalis [47] . Probably as a consequence of this metabolic parasitism, N. equitans has a drastically reduced genome size of only 0.5 megabases and thus depends entirely on its host for provisioning essential metabolites such as lipids, nucleotides, amino acids, and cofactors [48] . Interestingly, membranous structures connect host and symbiont and N. equitans obtains its amino acids from I. hospitalis [49] , which strikingly parallels the observations of our study. Also the recent observation that a shortage of nutrients seems to trigger an exchange of cytoplasmic constituents between cocultured cells of Desulfovibrio vulgaris and Clostridium acetobutylicum [50] corroborates the interpretation that bacteria may commonly establish direct cell-cell connections to counter nutritional stress. Several other examples have been documented, in which bacteria and/or archaea engage in obligate, metabolic interactions [51] , [52] —virtually all of which rely on close, physical associations between interacting partners. A direct intercellular transfer via nanotubes likely minimizes the loss of a given compound by diffusion, thereby reducing the physiological costs of producing the metabolite. Thus, nanotube-mediated cross-feeding is likely most relevant in nutrient-limiting or aqueous environments, whereas a diffusion of metabolites via the cell external environment should be more prevalent in nutrient-rich habitats, such as milk [53] , or when the exchanged metabolite is released in sufficiently high concentrations (for example, as a metabolic by-product [54] ). Furthermore, also for cells that are located within a close physical proximity such as a bacterial biofilm, it may be more efficient to transfer metabolites by diffusion [9] than to activate a contact-dependent transfer mechanism. However, it remains to be determined how intercellular networks affect the growth and metabolism of the cells involved, as well as which ecological factors favour their establishment. Theory predicts for a population of cells that perform two vital functions that, phenotypic specialists should emerge when their cumulative costs are less than the cost for one cell to perform both tasks [55] . Indeed, analysing cocultures of two E. coli genotypes that both required a different amino acid to grow, yet produced increased amounts of others, revealed a significant fitness advantage of cooperative cross-feeding relative to prototrophic WT cells [56] . Especially, the tremendous fitness advantage auxotrophic bacteria gain when the required metabolite is supplied externally [56] , [57] , [58] should exert a strong selection pressure that favours cross-feeding of essential metabolites among bacterial cells. The enormous variation in gene content that is commonly found among different genomes of E. coli [59] , [60] , together with the observation that often seemingly essential biosynthetic functions are lost [56] may reflect the ability of E. coli to compensate its metabolic deficiencies by connecting to other cells. Our discovery that bacteria utilize intercellular connections to exchange nutrients and thus complement each other’s metabolic requirements has significant implications for microbial ecology and physiology. The possibility that by connecting via nanotubes two or more bacterial cells can significantly extend their biochemical repertoire without the need for genetic change, suggests bacteria may function as multicellular, interconnected entities rather than as individual, physiologically autonomous units. Strains and plasmids Genetic targets, which would lead to metabolic auxotrophies for His and Trp (that is, hisD and trpB ) or an overproduction of His and Trp (that is, hisL and trpR ) upon deletion from the genomes of Acinetobacter baylyi ADP1 and Escherichia coli BW25113 were identified using the KEGG pathway database [61] . Acinetobacter baylyi ADP1 deletion mutants were constructed as described [62] . In brief, linear constructs of the kanamycin cassette with 5′-overhangs homologous to the insertion site were produced by PCR. For this, DNA of the plasmid pKD4 (ref. 63 ) was used as a template to amplify the kanamycin resistance cassette ( Supplementary Table 1 ). Upstream and downstream regions homologous to hisD , trpB , hisL, and trpR were amplified using primers with a 5′-extension that was complementary to the primers used to amplify the kanamycin cassette ( Supplementary Table 1 ). The three resulting products were combined by PCR to obtain the kanamycin cassette fused to the upstream and downstream homologous overhangs. Natural competence of A. baylyi was utilized to transform the linear fragments into the WT. Transformation was done by diluting 20 μl of a 16-h-old culture grown in LB medium. This diluted culture was incubated at 30 °C with shaking. Fifty μl PCR mix containing the deletion cassette was added to this culture and incubated at 30 °C with shaking for 2 h. Finally, the culture volume was concentrated to 100 μl, plated on LB agar plates containing kanamycin, and incubated at 30 °C for colonies to appear. To construct double-deletion mutants, the kanamycin resistance cassette was removed from the receiver’s genome. For this, upstream and downstream regions homologous to hisD , trpB , hisL, and trpR were amplified using primers with a 5′-extension that were complementary to each other ( Supplementary Table 1 ). E. coli BW25113 (ref. 64 ) was used as WT, into which deletion alleles from existing single-gene deletion mutants [64] were introduced by P1 transduction [65] . Double-deletion mutants were constructed using auxotrophic mutants as receiver and amino acid overproducing mutants as donor strains. For this, the kanamycin resistance cassette was removed from the receiver’s genome as described [63] . The cytoplasm of all mutant and WT strains were individually labelled with either pJBA24- egfp [24] or pJBA24- mCherry —two plasmids that constitutively express the ampicillin resistance gene bla , as well as a green (EGFP) or red (mCherry) fluorescent protein, respectively. pJBA24- mCherry was constructed by PCR amplifying mCherry using pFPV- mCherry [66] as a template and oligonucleotide primers mCherry-SphI (5′-ATATA GCATGC TGAGCAAGGGCGAG-3′) and mCherry-HindIII (5′-CTCTC AAGCTT ACTTGTACAGCTCGTCCATG-3′) (restriction sites are underlined). The resulting amplicon was digested with SphI and HindIII, and the mCherry -containing fragment ligated between an artificial ribosomal-binding site II (RBSII) and transcriptional terminators T 0 and T 1 of pJBA24 (ref. 67 ). Finally, all strains were transformed using either plasmid. All strains and plasmids used are listed in Supplementary Table 2 . Culture conditions and general procedures In all experiments, cells were grown in minimal medium for Azospirillium brasilense (MMAB) [68] without biotin, using fructose instead of malate as a carbon source. The required amino acids (that is, His and Trp) were supplemented singly or together if necessary (100 μM each). Replicate precultures were started with individual colonies picked from freshly streaked LB agar plates that have been incubated for 24 h. The next morning, precultures were diluted to an optical density (OD) 600 nm of 0.1 and subsequently 10 μl (~10 5 CFUs) were used to inoculate 1 ml MMAB medium. Amino acids in the abovementioned concentration were added to the MMAB medium as specified. All cultures were incubated at 30 °C for 24 h under shaking conditions (230 r.p.m,) in 96-deep-well plates (max. volume: 2 ml, Thermo Scientific Nunc) or (100 r.p.m.) in ‘Nurmikko cells’ (see ‘Population separation experiment’ below). Both the EGFP- and the mCherry-labelled variants of the focal genotypes were used in all experiments, unless specified otherwise. Antibiotics were used at the following concentrations: kanamycin 50 μg ml −1 and ampicillin 100 μg ml −1 . Supplementation experiment To identify whether auxotrophs and cross-feeders of both species required amino acids to grow, the corresponding strains were cultivated in 1 ml of unsupplemented or amino acid-containing MMAB medium (one amino acid). Cultures were plated on LB agar plates at 0 h and after 24 h, and the number of CFUs quantified. This experiment was replicated eight times. Amino acid quantification using biosensors The two amino acid auxotrophic E. coli strains ΔhisD and ΔtrpB were used as biosensors [24] to determine the production levels of His and Trp in growing cultures of WT, auxotrophs, overproducers, and cross-feeders. For this, precultures of all donor genotypes were inoculated (1:1 ratio) together with one of the two auxotrophs in 1 ml of MMAB medium. After 24 h, the population size of auxotrophs was determined by plating cocultures on LB agar plates that did or did not contain kanamycin. This experiment was replicated eight times per biosensor–donor combination. Amino acid quantification by liquid chromatography The amount of His and Trp the two cross-feeding genotypes of both A. baylyi and E. coli released during 24 h of growth in the external environment was quantified by liquid chromatography (LC). For this, eight replicate populations of all EGFP-labelled strains were grown separately in 1 ml MMAB medium containing either His or Trp (100 μM). After incubation, cultures were centrifuged (3,800 g for 20 min) and the supernatant immediately used for amino acid measurements. Histidine analysis was performed by reversed-phase high-performance LC on an Agilent 1100 HPLC system (Agilent Technologies, Böblingen, Germany) on a XDB-C18 (50 × 4.6 mm, 1.8 μm, Agilent Technologies) column with o -phtaldialdehyde-mercaptoethanol (OPA) pre-column derivatization. Each sample was pre-mixed with sodium borate buffer (0.5 M, pH 11) to a final volume of 100 μl. Derivatization was performed automatically by an Agilent 1100 autosampler (Agilent Technologies) that added 30 μl of a mixture of OPA (85 mM) and β-mercaptoethanol (130 mM) to the sample, incubated it for 2 min at room temperature and loaded 30 μl onto the column. The mobile phase consisted of a mixture of solvent A (10 mM ammonium acetate) and solvent B (acetonitrile). In the beginning, 10% of solution B was used, which rose to 20% in the course of 10 min. The flow rate was set to 0.8 ml min −1 . After 10 min, the mobile phase was switched to 100% solvent B for 4 min. After that the column was reconstituted for 3 min with 10% of solvent B before the next analysis cycle started. The amino acid-OPA derivatives were quantified using a fluorescence detector (Ex: 340 nm, Em: 445 nm). The calibration was done in the same way using a histidine standard in concentrations ranging from 0.005 to 0.05 μM. For tryptophan analysis, supernatant samples were diluted in a ratio of 1:10 (v:v) in water containing the 13 C, 15 N-labelled amino acid mix (Isotec, Miamisburg, OH, USA) and directly analysed by LC/MS/MS. The analysis method was modified from a protocol described by Jander et al. [69] . Chromatography was performed on an Agilent 1200 HPLC system (Agilent Technologies). Separation was achieved on a Zorbax Eclipse XDB-C18 column (50 × 4.6 mm, 1.8 μm, Agilent Technologies). Formic acid (0.05%) in water and acetonitrile were employed as mobile phases A and B, respectively. The elution profile was: 0–1 min, 3% B in A; 1–2.7 min, 3–100% B in A; 2.7–3 min, 100% B and 3.1–6 min, 3% B in A. The mobile phase flow rate was 1.1 ml min −1 . The column temperature was maintained at 25 °C. The LC was coupled to an API 3200 tandem mass spectrometer (Applied Biosystems, Darmstadt, Germany) equipped with a Turbospray ion source operated in positive ionization mode. The ionspray voltage was maintained at 5,500 eV. The turbo gas temperature was set at 700 °C. Nebulizing gas was set at 70 psi, curtain gas at 35 psi, heating gas at 70 psi, and collision gas at 2 psi. Multiple reaction monitoring was used to monitor analyte parent ion→product ion. Both Q1 and Q3 quadrupoles were maintained at unit resolution. Analyst 1.5 software (Applied Biosystems) was used for data acquisition and processing. All samples were spiked with 13 C, 15 N-labelled amino acids (algal amino acids 13 C, 15 N, Isotec) at a concentration of 10 μg of the mix per ml. Trp was quantified using 13 C, 15 N-Phe as internal standard applying a response factor of 0.42. Population separation experiment To determine whether physically separating cross-feeding genotypes prevents the reciprocal exchange of amino acids, a device was designed and constructed ( Supplementary Fig. 2 ) that allowed to separate two populations of bacterial cells with a membrane filter (0.2 μm, polyethersulfone, Pall GmbH, Germany). We named the device ‘Nurmikko cell’ after Veikko Nurmikko, a Finnish biochemist who developed a similar apparatus in 1957 (ref. 70 ). Pairs of cross-feeders were inoculated (1:1 ratio) in separate growth chambers of a Nurmikko cell (total volume: 8 ml), which were or were not separated by a filter membrane. Each combination (that is, pair of cross-feeder with or without filter) was replicated four times. The entire assembly was incubated at 30 °C for 24 h under shaking conditions (100 r.p.m.). The density of each cross-feeding partner was determined at the onset of the experiment and after 24 h by plating on MMAB plates containing selective amino acids (His or Trp). To test whether the membrane filter can hinder the diffusion of amino acids between two growth chambers of a Nurmikko cell ( Supplementary Fig. 2 ), each labelled variant of the individual cross-feeding strains was inoculated in one side of a Nurmikko cell. Afterwards, 80 μl of a 10-mM amino acid solution the genotype required for growth (that is, His or Trp) was supplemented either into the same growth chamber or, alternatively, across the filter membrane (final amino acid concentration: 100 μM). Cultures were incubated as before and plated on LB agar plates to estimate CFU counts at 0 h and after 24 h. This experiment was replicated four times. A control experiment was performed to test whether the growth of unseparated cross-feeders could be explained by a release of amino acids into the external growth environment. For this, the amount of His and Trp released by the GFP-labelled variants of the cross-feeding mutants of both species during 24 h of growth was determined by LC. Then, cross-feeding genotypes were cultivated for 24 h in saturating concentrations of either His or Trp (that is, 100 μM), a concentration that significantly exceeded the amounts cross-feeding genotypes would have produced during 24 h of growth (that is, 0.5 μM), or unsupplemented MMAB medium. After 0 and 24 h, cultures were plated on unsupplemented and kanamycin-containing LB agar plates and the number of CFUs was determined. This experiment was replicated eight times. Plasmid transfer experiment To determine whether plasmids are transferred between cells, pairs of cross-feeding genotypes within E. coli and two combinations of A. baylyi and E. coli were co-inoculated (1:1 ratio) in MMAB medium. However, only one of the two cross-feeding genotypes was labelled with the pJBA24- egfp plasmid, which also expressed ampicillin resistance (that is, bla gene). The population density of each cross-feeder was determined after 0 and 24 h by plating dilution series of vortexed cocultures on MMAB agar plates that contained either His or Trp, and the frequency of plasmid carriage was quantified by supplementing the amino acid-containing agar plates with ampicillin or no antibiotic as control. The proportion of EGFP-labelled cells at 0 h and after 24 h in each of the cocultures was determined by flow cytometry. This experiment was replicated three times. Flow cytometry The proportion of mCherry-, EGFP- and double-labelled cells (that is, cells containing both EGFP and mCherry) within a given coculture was determined by flow cytometry. To this end, cells were excited at 488 nm by a blue solid-state laser at 20 mW and at 561 nm by a yellow solid-state laser at 100 mW using a Partec CyFlow Space flow cytometer (Partec GmbH, Germany). Green and red fluorescence was detected at 536 nm (FL1) and 610 nm (FL3), respectively. Non-fluorescent E. coli WT culture was used as control to set the gates for EGFP- and mCherry-positive cells. Data acquisition and analysis was done using the FlowMax software (Partec GmbH). Flow cytometric analysis of cytoplasmic protein transfer Pairs of cross-feeding genotypes, whose cytoplasms were differentially labelled with a plasmid containing either egfp or mCherry were co-inoculated (1:1 ratio) in 1 ml MMAB medium. After 24 h, cocultures were diluted to OD 600 nm 0.01 and 20 μl of this culture transferred to 1 ml of fresh MMAB medium. Cocultures were sampled after 0, 12, 24 and 48 h and the number of single- and double-labelled cells was determined by flow cytometry. This experiment was replicated eight times. The same experiment was repeated with all three combinations of cross-feeders within E. coli and between A. baylyi and E. coli , yet this time cocultures were sampled at a much finer temporal resolution, namely after 0, 3, 6, 9, 12, 14, 15, 16, 17, 18, 19, 20, 22, 24 and 48 h, and the number of single- and double-labelled cells was determined as before. This experiment was replicated eight times. Two control experiments were performed to verify whether in the flow cytometrical measurements, double-labelled cells result from the sticking together of two individually labelled cells. First, the proportion of double-labelled cells was determined at 0 and at 24 h after applying no treatment, vortexing for 1 min or treating cells with a commercially available cell dissociation solution (FACSmax, Genlantis, USA). This experiment was replicated eight times. Second, the FSC of all double cells within a given coculture, as well as of E. coli WT labelled with pJBA24- egfp was determined after 24 h. In addition, the FSC of 1- and 2-μm-diameter microspheres (Molecular probes Inc., USA) was quantified. These measurements were replicated six times. The effect of amino acid availability on the exchange of cytoplasmic constituents between cross-feeding genotypes was determined for all pairs of double-deletion mutants, except the intraspecific comparison within A. baylyi . All cross-feeders were individually precultured and after 24 h diluted to an OD 600 nm of 0.01. Ten μl of these dilutions were used to co-inoculate two cross-feeding genotypes (1:1 ratio) in 1 ml of MMAB medium. After 24 h, the proportion of double-labelled cells in all cocultures was analysed by flow cytometry. This experiment was repeated four times. The role of the amino acid auxotrophy- or overproduction-causing mutations for inducing the nanotube-mediated exchange of cytoplasmic constituents was investigated by coculturing all possible pairs of EGFP- and mCherry-labelled variants of WTs, auxotrophs, overproducers and cross-feeders of both species, as described before. After 24 h, the percentage of double-labelled cells was quantified by flow cytometry. This experiment was replicated four times. Autofluorescence of EGFP- and mCherry-expressing cells To confirm that EGFP- and mCherry-labelled cells fluoresce only at the expected wavelength, all cross-feeding genotypes expressing EGFP and mCherry were inoculated in MMAB medium supplemented with ampicillin, as well as the required amino acid (His and Trp). After 0, 24 and 48 h of incubation, the emission levels of red and green fluorescence was determined by flow cytometry in all eight replicate cultures. Fitness of EGFP- and mCherry-expressing cells Competitive fitness experiments between the two variants of the same cross-feeding genotype labelled with either the pJBA24- egfp or pJBA24- mCherry plasmid were co-inoculated in equal densities (~10 5 CFUs ml −1 each) in MMAB medium containing the required amino acid (that is, His or Trp), which was supplemented with ampicillin. After 0 and 24 h, CFU numbers were determined by plating on LB plates with ampicillin. EGFP- and mCherry-expressing cells were distinguished based on the colour colonies developed on LB agar plates (mCherry: pink; EGFP: green). Competitive fitness of the differentially labelled cross-feeding genotypes was determined by calculating the Malthusian parameter ( M ) of both genotypes: M =(ln ( N f / N i )/24), where N i is initial number of CFUs at 0 h and N f is the final CFU count after 24 h [71] . Relative fitness was calculated as the ratio of Malthusian parameters. This experiment was replicated four times. Cytoplasmic exchange in shaken and static conditions To test whether static culture conditions enhance the cytoplasmic constituents, pairs of cross-feeding strains, whose cytoplasms were differentially labelled with EGFP and mCherry, were co-inoculated (1:1 ratio) in 1 ml MMAB medium. These cocultures were either incubated at 30 °C under shaken conditions (230 r.p.m.) or in unshaken, static conditions. Cocultures were sampled after 0 and 24 h and the numbers of single- and double-labelled cells were determined by flow cytometry, and the number of CFUs quantified by plating on LB agar plates. This experiment was replicated three times. Fluorescence microscopy The emission of red and green fluorescence from individual cells was confirmed by fluorescence microscopy. For this, all possible pairs of EGFP- or mCherry-labelled cross-feeders were co-inoculated (1:1 ratio) in 1 ml of unsupplemented or amino acid-supplemented MMAB medium (that is, both His and Trp). After 24 h, samples were drawn and a drop was fixed on a microscopy slide. An Axio Imager Z1 Zeiss microscope (Carl Zeiss AG, Jena, Germany) was used to observe bacterial cells. Images were analysed using the software AxioVision LE Rel. 4.4 (Carl Zeiss AG). Fluorescence time-lapse microscopy Cells were grown in liquid medium as above and thereby allowed to induce nanotube formation. Subsequently, cells were spread on a gel pad 1.5% Ultra Pure Agarose (Invitrogen, Darmstadt, Germany). Images were taken on an inverted epi-fluorescence microscope (Delta Vision Elite Imaging System, GE Healthcare) using a × 100, 1.4 numerical apperture UPlanSApo objective (Olympus) and a PCS Edge sCMOS camera. Focus was maintained using the Ultimate Focus system. Samples were imaged every 2 min using brightfield and fluorescence illumination, respectively, by applying the following filter and exposure conditions: GFP (475/28 nm, 525/50 nm) for 25 ms at 5% intensity, mCherry (575/25 nm 632/60 nm) for 15 ms at 10% and POL (5 ms, 32%). Under these exposure conditions, single-labelled cells did not show fluorescence in the respective other channel. For display, image stacks were split into three channels (red, green, and grey), converted into single images and merged for a specific time point using the Fiji software [72] . To visualize nanotubes, brightness and contrast settings were adjusted and a local contrast enhancement (CLAHE) followed by smoothening was applied in Fiji [72] to obtain the final output ( Fig. 6a ). Fluorescence intensities of a given cell were determined by first splitting the image into the different channels (green and red). Next, fluorescent images were individually merged with a brightfield microscopic image to determine the cell outline. A line was then mapped across the cell and a plot profile of 30 grey values was generated. Subsequently, the line was shifted to a region with no cells in a radius of 20 μm from the focal cell to determine the background fluorescence. For calculation of final values, the average background fluorescence was subtracted from the fluorescence intensities (grey values) of the cells. Fluorescence intensities were determined for each of the 17 frames (interval: 2 min). Lipid dye experiment To determine whether nanotubes were lipid-based, 5 μl of Vybrant DiO Cell-Labelling Solution (Invitrogen) were added to 1 ml of a 9-h-old coculture of the interspecific cross-feeding consortium, of which both strains were labelled with the mCherry-expressing plasmid. After that, cells were incubated for 30 min in the dark at 30 °C and subsequently imaged on agar pads using inverted epi-fluorescence microscopy as described above. Visualization of membrane structures was improved by applying a nonlinear histogram adjustment to fluorescence images using Fiji software [72] . Scanning electron microscopy Cross-feeding strains were co-inoculated (1:1 ratio) in 1 ml of unsupplemented or amino acid-supplemented MMAB medium (that is, both His and Trp), and after 24 h of growth, sedimented on poly- L -lysine-coated (Sigma-Aldrich) glass coverslips. Samples were fixed for 1 h with 2.5% glutaraldehyde in sodium cacodylate buffer (0.1 M, pH 7.0) and dehydrated with ethanol in serially increased concentration, followed by critical point drying in a Leica EM CPD300 Automated Critical Point Dryer (Leica, Germany). Then, samples were sputter-coated with gold (layer 25 nm) in a BAL-TEC SCD005 Sputter Coater (BAL-TEC, Liechtenstein) and analysed at different magnifications with a LEO 1530 Gemini field emission scanning electron microscope (Carl Zeiss) at 5 kV acceleration voltage and a working distance of 5 mm using an in-lense secondary electron detector. Statistical analysis Growth of a given (co-) culture during 24 h was expressed as ‘cell count’, which refers to the number of CFUs reached after 24 h minus the CFU number at 0 h. ‘Net cell count’ is the cell count a given strain reached in coculture minus its cell count in monoculture. Statistical differences between two experimental groups were identified using paired t -tests. Wilcoxon signed rank tests were performed when variances were inhomogeneous. Univariate analyses of variance followed by a LSD post hoc test were used to compare more than two experimental groups. Statistical differences in the proportion of EGFP-labelled cells at 0 and 24 h were identified using a replicated G -test of goodness-of-fit. One-sample t -tests were performed to test whether the competitive fitness of differentially labelled cross-feeding genotypes deviated significantly from 1 (that is, no fitness difference). Accession codes: The unprocessed raw image files used to compile Supplementary Movie 1 and generate Fig. 7b,c are available at the Dryad Digital Repository ( http://doi.org/10.5061/dryad.ds68k ). How to cite this article: Pande, S. et al. Metabolic cross-feeding via intercellular nanotubes among bacteria. Nat. Commun. 6:6238 doi: 10.1038/ncomms7238 (2015).